New diluted ferromagnetic semiconductor with Curie temperature up to 180 K and isostructural to the ‘122’ iron-based superconductors Diluted magnetic semiconductors have received much attention due to their potential applications for spintronics devices. A prototypical system (Ga,Mn)As has been widely studied since the 1990s. The simultaneous spin and charge doping via hetero-valent (Ga 3+ ,Mn 2+ ) substitution, however, resulted in severely limited solubility without availability of bulk specimens. Here we report the synthesis of a new diluted magnetic semiconductor (Ba 1− x K x )(Zn 1− y Mn y ) 2 As 2 , which is isostructural to the 122 iron-based superconductors with the tetragonal ThCr 2 Si 2 (122) structure. Holes are doped via (Ba 2+ , K 1+ ) replacements, while spins via isovalent (Zn 2+ ,Mn 2+ ) substitutions. Bulk samples with x =0.1−0.3 and y =0.05−0.15 exhibit ferromagnetic order with T C up to 180 K, which is comparable to the highest T C for (Ga,Mn)As and significantly enhanced from T C up to 50 K of the ‘111’-based Li(Zn,Mn)As. Moreover, ferromagnetic (Ba,K)(Zn,Mn) 2 As 2 shares the same 122 crystal structure with semiconducting BaZn 2 As 2 , antiferromagnetic BaMn 2 As 2 and superconducting (Ba,K)Fe 2 As 2 , which makes them promising for the development of multilayer functional devices. Diluted Magnetic Semiconductors (DMSs) have received much attention due to their potential applications for spin-sensitive electronics (spintronics) [1] , [2] , [3] , [4] , [5] . DMS systems are produced by doping semiconductors with magnetic metal elements. In typical systems based on III–V semiconductors, such as (Ga,Mn)As, (In,Mn)As and (Ga,Mn)N, substitution of divalent Mn atoms into trivalent Ga (or In) sites leads to severely limited chemical solubility, resulting in metastable specimens only available as epitaxial thin films. The hetero-valent substitution, which simultaneously dopes both hole carriers and magnetic atoms, makes it difficult to individually control charge and spin concentrations for better tuning of quantum freedom. Following a theoretical proposal by Masek et al . [6] , a new system Li(Zn,Mn)As was recently synthesized by Deng et al . [7] based on the I–II–V semiconductor LiZnAs, showing a Curie temperature up to T C =50 K. In this system, charges are doped via off-stoichiometry of Li concentrations, while spins by the isovalent (Zn 2+ ,Mn 2+ ) substitutions. Although Li(Zn,Mn)As was a ferromagnetic DMS of a new type having a few distinct advantages over (Ga,Mn)As, the upper limit of currently achievable T C has been significantly lower than that in (Ga,Mn)As [2] , [7] . BaZn 2 As 2 [8] is a semiconductor synthetized at high temperature (>900 °C) with the tetragonal ThCr 2 Si 2 crystal structure (shown in Fig. 1a ), identical to that of BaFe 2 As 2 ( [9] ), BaMn 2 As 2 ( [10] , [11] ) and (Ba,K)Mn 2 As 2 ( [12] ). (Ba,K)Fe 2 As 2 ( [9] , [13] ) is a classic member of the ‘122’ type iron pnictide superconductors with transition temperature up to 38 K, whereas BaMn 2 As 2 is an antiferromagnet with T N ~625 K (refs 11 , 12 ). It is noted that the stable phase at room temperature of BaZn 2 As 2 crystallizes into a different orthorhombic structure with space group Pnma [8] ( Supplementary Fig. S1 ). However, we found that 10% of K or Mn doping dramatically stabilizes the tetragonal ThCr 2 Si 2 structure at room temperature down to T =3.5 K ( Supplementary Fig. S2 ). Here we report the synthesis of a new ferromagnetic DMS (Ba,K)(Zn,Mn) 2 As 2 system, which shares the same ‘122’ structure with (Ba,K)Fe 2 As 2 and (Ba,K)Mn 2 As 2 . 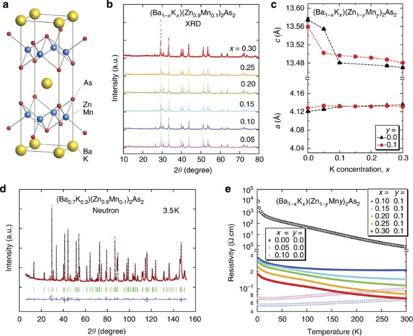Figure 1: Structural and electrical properties of (Ba,K)(Zn,Mn)2As2 (a) Crystal structure of (Ba,K)(Zn,Mn)2As2belonging to tetragonal ThCr2Si2structure. (b) X-ray diffraction (XRD) pattern of (Ba1−xKx)(Zn0.9Mn0.1)2As2with several K concentrationsxtaken at room temperature. (c)caxis andaaxis lattice constants obtained from XRD. (d) Neutron diffraction pattern from powder specimen of (Ba1−xKx)(Zn0.9Mn0.1)2As2withx=0.3 shown with Rietveld analyses. (e) Resistivity of (Ba1−xKx)(Zn1−yMny)2As2for the pure Zn (y=0) and Mn 10% (y=0.1) systems with several different charge doping levelsx. Note that the vertical axis for the pure BaZn2As2is very different from that for other specimen. Via (Ba,K) substitution to dope hole carriers and (Zn,Mn) substitution to supply magnetic moments, samples with 5–15% Mn doping exhibit ferromagnetic order with T C up to 180 K. Figure 1: Structural and electrical properties of (Ba,K)(Zn,Mn) 2 As 2 ( a ) Crystal structure of (Ba,K)(Zn,Mn) 2 As 2 belonging to tetragonal ThCr 2 Si 2 structure. ( b ) X-ray diffraction (XRD) pattern of (Ba 1− x K x )(Zn 0.9 Mn 0.1 ) 2 As 2 with several K concentrations x taken at room temperature. ( c ) c axis and a axis lattice constants obtained from XRD. ( d ) Neutron diffraction pattern from powder specimen of (Ba 1− x K x )(Zn 0.9 Mn 0.1 ) 2 As 2 with x =0.3 shown with Rietveld analyses. ( e ) Resistivity of (Ba 1− x K x )(Zn 1− y Mn y ) 2 As 2 for the pure Zn ( y =0) and Mn 10% ( y =0.1) systems with several different charge doping levels x . Note that the vertical axis for the pure BaZn 2 As 2 is very different from that for other specimen. Full size image Synthesis and structural characterization Polycrystalline specimens of (Ba,K)(Zn,Mn) 2 As 2 were synthesized using the arc-melting solid-state reaction method similar to that described in ref. 7 . Details of the synthesis and instruments used for characterization are described in the Methods section. Figure 1b shows the X-ray diffraction results of (Ba 1− x K x )(Zn 0.9 Mn 0.1 ) 2 As 2 for x =0.05, 0.1, 0.15, 0.2, 0.25 and 0.3, respectively. Patterns with a 2 θ range (10°–80°) were collected, and the least-squares method was used to determine the lattice parameters of all polycrystalline samples, as shown in Fig. 1c . Compared with the lattice parameters a =4.121 Å and c =13.575 Å of BaZn 2 As 2 , the a axis expanded and the c axis shrank in (Ba 1− x K x )Zn 2 As 2 . For compounds with Mn 10%, (Ba 1− x K x )(Zn 0.9 Mn 0.1 ) 2 As 2 , the c axis has similar tendency with Mn free (Ba 1− x K x )Zn 2 As 2 , while the a axis does not show obvious variation with doping. These results indicate successful solid solutions of K and Mn. Further structural studies have been made by neutron diffraction measurements from a powder specimen of (Ba 1− x K x )(Zn 0.9 Mn 0.1 ) 2 As 2 with x ~0.3 at the FRM-II reactor in TU Munich. The powder diffraction pattern, shown in Fig. 1d , fitted well to the structure found by X-rays, and the contrasting neutron scattering length of Mn and Zn allowed us to confirm random substitution of Mn atoms in Zn sites. The residuals of the Rietveld analysis were about 4–5%. There was no structural phase transition below T ~300 K, which is in contrast to the case of antiferromagnetic (Ba,K)Fe 2 As 2 ( [9] ). Because of the small average moment size (average 0.1 Bohr magneton per Zn/Mn site) and limited neutron intensity, we could not detect a conclusive signal from ferromagnetic spins below T C . Resistivity Resistivity measurements shown in Fig. 1e indicate that BaZn 2 As 2 is a semiconductor. Doping K atoms into Ba sites introduces hole carriers, leading to metallic behaviour in (Ba,K)Zn 2 As 2 . The resistivity curves of (Ba 1− x K x )(Zn 0.9 Mn 0.1 ) 2 As 2 , for selected values of x up to 0.3, exhibit a small increase at low temperatures due presumably to spin scattering of carriers caused by Mn dopants. This variation of resistivity, similar to that of (Ga,Mn)N (ref. 14 ), is often observed in heavily doped semiconductors. Strictly metallic behaviour (with monotonic decrease of resistivity with decreasing temperatures) is not a precondition of having a ferromagnetic coupling between Mn moments mediated by RKKY interaction, as discussed in refs 1 and 15 . 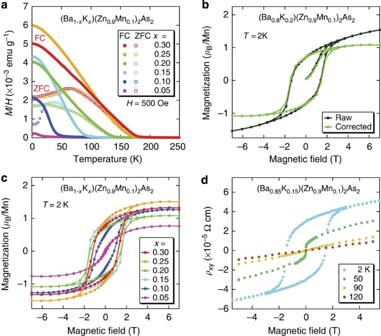Figure 2: Magnetic properties of (Ba,K)(Zn,Mn)2As2 (a) DC magnetization measured inH=500 G in (Ba1−xKx)(Zn0.9Mn0.1)2As2with several different charge doping levelsx, with ZFC and FC procedures. (b) Magnetic hysteresis curveM(H), measured in the external fieldHup to 7 T, showing initial magnetization curve and subtraction of a small T-linear contribution. (c)M(H) curves after field training and subtraction of the paramagnetic component measured in (Ba1−xKx)(Zn0.9Mn0.1)2As with several different charge doping levelsx. (d) Hall effect results from a sintered specimen of (Ba1−xKx)(Zn0.9Mn0.1)2As2with the charge doping level ofx=0.15 havingTC~90 K. Anomalous Hall effect and a very small coercive field is seen atT=50 K near the history-dependence temperatureTHist, while a large coercive field is seen atT=2 K. Magnetization, Hall effect and hysteresis Figure 2a shows temperature dependence of magnetization in zero-field-cooling (ZFC) and field-cooling (FC) procedures under 500 Oe for (Ba 1− x K x )(Zn 0.9 Mn 0.1 ) 2 As 2 specimens with x =0.05, 0.1, 0.15, 0.2, 0.25 and 0.3, respectively. Clear signatures of ferromagnetic order are seen in the curves, with corresponding critical temperature T C =5 K, 40 K, 90 K, 135 K, 170 K and 180 K, respectively. Above T C , the samples are paramagnetic and the susceptibility χ ( T ) can be fitted to the Curie–Weiss formula with an effective paramagnetic moment ~5 μ B per Mn 2+ . The hysteresis curves M ( H ) at T =2 K in Fig. 2b exhibit an initial increase from H =0 state achieved by ZFC procedure, and a small H-linear component, which is presumably due to remaining paramagnetic spins and/or field-induced polarization. By subtracting this small T -linear component, we obtain the M ( H ) curves of (Ba 1−x K x )(Zn 0.9 Mn 0.1 ) 2 As 2 at T =2 K shown in Fig. 2c . The saturation moment of 1~2 μ B per Mn atom is comparable with that of (Ga,Mn)As [1] and Li(Zn,Mn)As [7] . Figure 2: Magnetic properties of (Ba,K)(Zn,Mn) 2 As 2 ( a ) DC magnetization measured in H =500 G in (Ba 1− x K x )(Zn 0.9 Mn 0.1 ) 2 As 2 with several different charge doping levels x , with ZFC and FC procedures. ( b ) Magnetic hysteresis curve M ( H ), measured in the external field H up to 7 T, showing initial magnetization curve and subtraction of a small T-linear contribution. ( c ) M ( H ) curves after field training and subtraction of the paramagnetic component measured in (Ba 1− x K x )(Zn 0.9 Mn 0.1 ) 2 As with several different charge doping levels x . ( d ) Hall effect results from a sintered specimen of (Ba 1− x K x )(Zn 0.9 Mn 0.1 ) 2 As 2 with the charge doping level of x =0.15 having T C ~90 K. Anomalous Hall effect and a very small coercive field is seen at T =50 K near the history-dependence temperature T Hist , while a large coercive field is seen at T =2 K. Full size image The Hall effect measurements indicate that 10% (Ba,K) substitution in (Ba,K)Zn 2 As 2 results in hole concentration of 4.3 × 10 20 cm −3 , consistent within a factor of two with that obtained by assuming that each K atom introduces one hole to the system. In (Ba,K)(Zn,Mn) 2 As 2 , linear dependence of Hall resistivity with magnetic field is observed above T C . As shown in Fig. 2d for the x =0.15 and y =0.10 system, having T C =90 K, the Hall resistivity deviates from the linear dependence in low field at T C . In the ferromagnetic state below T C , the anomalous Hall effect is observed with a small coercive field ∼ 35 Oe in the temperature region between T C and the history-dependence temperature T Hist below which FC and ZFC susceptibility shows deviation. The small coercive field above T Hist will be helpful for spin manipulation. The deviation between the magnetization in FC and ZFC procedures in Fig. 2a and a large difference between the initial and the field-trained M ( H ) curves in Fig. 2b can be ascribed to a large coercive force demonstrated in Fig. 2c below T Hist . A very similar departure of ZFC and FC magnetization, associated with a coercive field~1 T, was observed in a well-known itinerant ferromagnet SrRuO 3 ( [16] , [17] ), which has a comparable T C ~160 K. The large coercive field at low temperatures in (Ba,K)(Zn,Mn) 2 As 2 is different from Li(Zn,Mn)As, which exhibits a small coercive field of~100 G in the entire temperature region [7] . The large temperature dependence of the coercive field in (Ba,K)(Zn,Mn) 2 As 2 opens a possibility of temperature tuning of anisotropy and stability of magnetic memory. Muon spin relaxation (MuSR) Using bulk polycrystalline specimens, we also performed positive MuSR measurements at Paul Scherrer Institute. 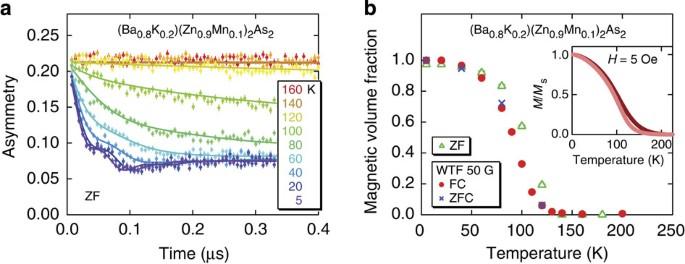Figure 3: MuSR measurements (a) ZF-MuSR time spectra obtained in polycrystalline specimen of (Ba0.8K0.2)(Zn0.9Mn0.1)2As2. The error bars represent statistical errors determined by the number of total muon decay events observed per each data. (b) Volume fraction of regions with static magnetic order, estimated by MuSR measurements in ZF and weak transverse field (WTF) of 50 G. No hysteresis is seen for WTF measurements with ZF cooling and field cooling in 500 G. Inset: DC magnetization results of the specimens used in MuSR measurements. Figure 3a shows the time spectra of the zero-field (ZF) MuSR on a (Ba 0.8 K 0.2 )(Zn 0.9 Mn 0.1 ) 2 As 2 specimen, which has T C ~140 K, as determined by magnetization (inset of Fig. 3b ). A sharp increase of the MuSR relaxation rate is seen with decreasing temperature below T C , and a highly-damped precession signal was observed below T ~40 K. The volume fraction of magnetically ordered state was estimated by using MuSR data in ZF and weak transverse field of 50 G as shown in Fig. 3b . The MuSR results indicate static magnetic order developing in the entire volume with a rather sharp onset below T C . Figure 3: MuSR measurements ( a ) ZF-MuSR time spectra obtained in polycrystalline specimen of (Ba 0.8 K 0.2 )(Zn 0.9 Mn 0.1 ) 2 As 2 . The error bars represent statistical errors determined by the number of total muon decay events observed per each data. ( b ) Volume fraction of regions with static magnetic order, estimated by MuSR measurements in ZF and weak transverse field (WTF) of 50 G. No hysteresis is seen for WTF measurements with ZF cooling and field cooling in 500 G. Inset: DC magnetization results of the specimens used in MuSR measurements. Full size image The ZF precession spectra in Fig. 3a at T =5 K and 20 K look very similar to those observed in the ferromagnetic SrRuO 3 by ZF-MuSR (see Fig. 7 of refs 18 and 19 ). Small oscillation amplitudes in both systems may be due to domain structures and spread of demagnetizing field in polycrystalline specimens. We also note that ZF-MuSR spectra did not show oscillation in ferromagnetic Li(Zn,Mn)As [7] and (Ga,Mn)As [15] . In all these DMS systems, random substitution of Mn at Zn or Ga sites generates a spatially random distribution of Mn moments, which makes the local field at the muon site highly random even in the ferromagnetic ground state. Because of this feature, ZF precession signals are strongly damped. In Table 1 , we summarize transition temperature T C determined by ZFC and FC magnetization, and the size of the ordered moment per Mn at T =2 K, obtained from the H =0 values of the M(H) curve after cycling the field to 7 T, for (Ba 1− x K x )(Zn 1− y Mn y ) 2 As 2 with the K concentration x up to 0.3 and Mn concentration y up to 0.15. The highest T C is obtained for x =0.3 and y =0.1. We notice a tendency for the reduction of the moment size with increasing Mn doping, which may result from competition between antiferromagnetic coupling of Mn moments in the nearest neighbour Zn sites and ferromagnetic coupling between Mn moments in more distant locations mediated by the doped hole carriers. This feature is common to (Ga,Mn)As and Li(Zn,Mn)As. Table 1 Transition temperature T C and the saturation moment M S ( H =0) at T =2 K after training in the external field of 7 T for Ba 1− x K x (Zn 1− y Mn y ) 2 As 2 with several different Mn spin doping levels y and hole charge doping levels x. Full size table Table 2 compares a few selected basic properties of the present compound with those of (Ga,Mn)As and Li(Zn,Mn)As. The present system is different from Li(Zn,Mn)As in several aspects: first, the currently available highest value of T C is more than three times higher in (Ba,K)(Zn,Mn) 2 As 2 than that in Li(Zn,Mn)As. Furthermore, the present system shows a very high coercive field at low temperatures. In addition, notable differences lie in crystal structures. The crystal structure of the ‘111’ DMS system Li(Zn,Mn)As, is different from that of the relevant antiferromagnet LiMnAs and also from superconducting LiFeAs, although they share common square-lattice As layers. In the present ‘122’ DMS ferromagnet (Ba,K)(Zn,Mn) 2 As 2 , semiconducting BaZn 2 As 2 , antiferromagnetic BaMn 2 As 2 and superconducting (Ba,K)Fe 2 As 2 all share the same crystal structure shown in Fig. 1a , except for a small orthorhombic distortion in (Ba,K)Fe 2 As 2 associated with antiferromagnetic order. Moreover, the lattice constants in the a-b plane match within about 5% as shown in Table 3 . These features could provide distinct advantages to the present system over the 111 DMS systems in attempts to generate functional devices based on junctions of various combinations of these states. Table 2 Selected properties of (Ga,Mn)As, Li(Zn,Mn)As and (Ba,K)(Zn,Mn) 2 As 2 . Full size table Table 3 Crystal structures and lattice constants of superconducting (Ba,K)Fe 2 As 2 , antiferromagnetic BaMn 2 As 2 , semiconducting BaZn 2 As 2 and ferromagnetic (Ba,K)(Zn,Mn) 2 As 2 . Full size table Possible research use of such junctions includes, for example, quantitative estimation of the carrier spin polarization and scattering strength via Andreev reflection at the DMS–superconductor interface [20] . In conclusion, we presented successful synthesis of a new ferromagnetic DMS system with T C up to 180 K developed over the entire volume. Availability of bulk specimens, independent spin and charge controls and perfect lattice matching with the 122 FeAs superconductors and relevant antiferromagnets make this promising system decisively different from the existing DMS systems based on the III–V semiconductors. Material synthesis Polycrystalline specimens of (Ba,K)(Zn,Mn) 2 As 2 were synthesized using the arc-melting solid-state reaction method similar to that described in ref. 7 . The starting materials, namely, precursors of BaAs, KAs, ZnAs, and high-purity Mn powders, were mixed according to the nominal composition of (Ba,K)(Zn,Mn) 2 As 2 . The mixture was sealed inside an evacuated tantalum tube that is, in turn, sealed inside an evacuated quartz tube. The mixture was heated until 750 °C at 3 °C min −1 . Then, the temperature was maintained for 20 h before it was slowly decreased to room temperature at a rate of 2 °C min −1 . Samples were characterized by X-ray powder diffraction with a Philips X'pert diffractometer using Cu K-edge radiation. The DC magnetic susceptibility was characterized using a superconducting quantum interference device magnetometer (Quantum Design, Inc.), whereas the electronic-transport were measured using a physical property-measuring system. Neutron powder diffraction measurements were performed at the FRM-II reactor in TU Munich using the SPODI spectrometer (for details of SPODI, see http://www.sciencedirect.com/science/article/pii/S0168900211021383 .) How to cite this article: Zhao, K. et al . New diluted ferromagnetic semiconductor with Curie temperature up to 180 K and isostructural to the ‘122’ iron-based superconductors. Nat. Commun. 4:1442 doi: 10.1038/ncomms2447 (2012).